Mouse strains to study cold-inducible beige progenitors and beige adipocyte formation and function Cold temperatures induce formation of beige adipocytes, which convert glucose and fatty acids to heat, and may increase energy expenditure, reduce adiposity and lower blood glucose. This therapeutic potential is unrealized, hindered by a dearth of genetic tools to fate map, track and manipulate beige progenitors and ‘beiging’. Here we examined 12 Cre/inducible Cre mouse strains that mark adipocyte, muscle and mural lineages, three proposed beige origins. Among these mouse strains, only those that marked perivascular mural cells tracked the cold-induced beige lineage. Two SMA-based strains, SMA-Cre ERT2 and SMA-rtTA, fate mapped into the majority of cold-induced beige adipocytes and SMA-marked progenitors appeared essential for beiging. Disruption of the potential of the SMA-tracked progenitors to form beige adipocytes was accompanied by an inability to maintain body temperature and by hyperglycaemia. Thus, SMA-engineered mice may be useful to track and manipulate beige progenitors, beige adipocyte formation and function. Cold temperatures and adrenergic agonists can stimulate the formation of multilocular brown adipocytes in white adipose depots [1] . These new brown adipocytes, referred to as ‘beige’ or ‘brite’ adipocytes, dissipate heat and consume glucose and fatty acids [2] , [3] . Because of these attributes, beige adipocytes hold therapeutic potential to combat obesity and diabetes [4] . However, the source of beige adipocytes remains controversial and transdifferentiation of unilocular white adipocytes to multilocular beige adipocytes has been a conventional notion [5] , [6] . This is exemplified in recent work of Granneman and colleagues [7] , indicating that cells marked by Adiponectin-Cre ERT2 ; red fluorescent protein (RFP), which include white adipocytes, can fate map into beige adipocytes after cold exposure. In contrast, work by Scherer and colleagues [8] and work from others have suggested a different source; some imply a myogenic ancestry [9] , [10] . Another alternative may be smooth muscle-like progenitors that express myosin heavy chain 11 ( Myh11 ), suggested by a recent cell marking/fate-mapping study by Spiegelman and colleagues [11] . Granneman and colleagues [12] have also identified a perivascular platelet-derived growth factor receptor-α ( PDGFRα )-positive cell as a possible source for β3 agonist-induced beige adipocytes. These studies resonate with previous proposals of a mural cell (for example, vascular smooth muscle cells and pericytes) origin for white adipose progenitors, pointing to potential commonality between white and beige adipocyte provenance [13] , [14] . Yet, Sidossis and Kajimura [15] recently highlighted that in lieu of seminal fate-mapping studies, the origin(s) of beige adipocytes is not well defined and many pieces to the puzzle are missing such as age, gender and location within the adipose depot where beige adipocytes form at room temperature and after cold exposure. These obscurities are critical roadblocks to manipulating these cellular furnaces for therapeutic ends. The Cre/loxP site-specific recombination system has provided insight into tissue development, homeostasis and function [16] . Although ‘straight’ Cre drivers can be useful, they are limited for fate mapping and progenitor identification, because it is difficult to know when and where the actions of the Cre driver occurred [17] . To ascertain this information requires an extensive search, throughout development and adulthood, to delineate the temporal and spatial expression pattern of the Cre driver. Another concern of straight Cre marking is that the Cre allele can be continually expressed or functional, and also that its expression can be activated during the differentiation process of the cell type of interest, masking progenitorship [18] . Together with the other issues, this often undermines the use of straight Cre strains for fate mapping. These issues have in part been overcome by modifications that provide temporal precision, such as the tamoxifen (TM)-inducible Cre ER/ERT2 or the inducible/suppressible Tet systems [19] , [20] . These inducible tools are just transiently active, principally during the period in which the inducers such as doxycycline (Dox) or TM are administered [19] , [20] . During this window, Cre is active and reporter expression is turned on, presumably only in Cre-expressing cells that can be scored and sometimes in a relatively straightforward manner. After induction and chase, reporter marking can be present in potential descendants, providing insight into lineage and fate [19] , [21] . Mice that contain such inducible genetic tools have allowed scientists to identify stem cells/progenitors and to delineate the roles of these cells in tissue development, homeostasis and function [14] , [22] . Here we examined various straight Cre ( Myf5-Cre, Myogenin-Cre and SM22-Cre ) and inducible Cre ( AdipoTrak-tTA-TRE-Cre , Adiponectin-Cre ERT2 , aP2-Cre ERT2 , Myh11-Cre ERT2 , NG2-Cre ERT2 , PDGFRα-Cre ERT2 , SMA-Cre ERT2 , SMA-rtTA-TRE-Cre and UCP1-Cre ERT2 ) mouse strains, integrating an indelible Cre-dependent Rosa26R RFP allele, to attempt to fate map beige progenitors and beiging in response to cold stimuli. We found that SMA-Cre ERT2 - and SMA-rtTA-driven reporters and endogenous smooth muscle actin (SMA) were expressed in mural cells in all white adipose depots. Endogenous SMA expression was not detected in mature white or beige adipocytes, or other cells in the depots, and the SMA reporters mirrored that pattern at room temperature (RT) pulse. However, cold exposure triggered an evolution of SMA-dependent reporter expression and fate mapping was present in ∼ 60–80% of cold-induced uncoupling protein 1 (UCP1)-positive multilocular beige adipocytes in subcutaneous and visceral adipose depots. This high percentage fate mapping was supported in necessity tests; SMA mural-resident progenitors appeared essential for cold-induced beiging and the resultant mice had impaired physiological and metabolic responses to cold temperatures. SMA-based tools may therefore be useful to track and manipulate beige adipocyte development, formation and function, as well as metabolism. Mural cell genetic tools fate map into beige adipocytes We analysed a variety of genetically modified mice that express Cre or inducible/suppressible forms of Cre in adipose, muscle and mural cell lineages for the potential to mark cold-induced beige adipocytes in either subcutaneous inguinal or visceral perigonadal adipose depots. To visualize Cre-dependent marking, we incorporated an indelible Rosa26R RFP (tdTomato) reporter allele that expresses RFP in Cre-expressing cells and in potential descendants [23] . RFP is well suited for cell-fate studies, as it is quite sensitive, can be directly visualized with fluorescence microscopy and is convenient for immunohistochemistry (IHC) and flow cytometry (quantification and isolation) [14] . We performed experiments on 2-month-old Cre- or Cre ERT2 -Rosa26R RFP marking mice that were randomly housed for 7 days in either cold temperature (6 °C), to induce the beiging phenomena, or RT (23 °C), to serve as a control ( Fig. 1a ). To determine whether cold exposure induced beige adipocytes derived from a Cre-marked source, we examined RFP fluorescence either from intact depots or from histological sections, the latter combined with UCP1 IHC to help define beige adipocytes [24] , [25] . Our rational for whole depot imaging was to provide an overview of potential effects and to assess whether reporter expression might, for example, show a cold-induced evolution from vascular marking into new adipose tissue expression, as such a change may indicate that the marked cells were an origin for the beige phenomena. Beiging was less prominent in visceral perigonadal adipose depots, consistent with many scientists’ observations [6] , [8] , [12] , [26] , but cold exposure did induce the formation of small islands of beige adipocytes within this depot from male mice. 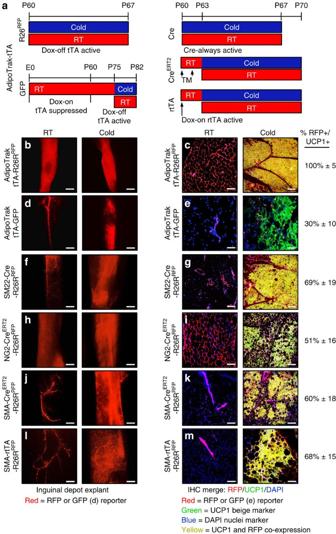Figure 1: Cre drivers with high beige adipocyte labelling. (a–m) Two-month-old male Cre mice (AdipoTrak-CreandSM22-Cre);R26RRFPmouse models (b,c,f,g) were maintained at RT (23 °C) or cold exposed (6 °C) for 7 days as shown ina. Subcutaneous inguinal adipose depot explants were imaged for direct RFP fluorescence or sectioned and immunostained for reporter (RFP, red) and UCP1 (green); co-expression (RFP+UCP1) is a yellow-gold hue. Cell nuclei were counterstained with DAPI (blue). Two-month-old male, inducible Cre mice (NG2-CreERT2;SMA-CreERT2andSMA-rtTA-TRE-Cre);R26RRFPmice (h–m) were administered one dose of TM on 2 consecutive days or administered Dox 3 days before experimentation. Mice were maintained at RT or cold exposed for 7 days as shown ina. Subcutaneous inguinal adipose depot explants were imaged or were sectioned and immunostained for reporter (RFP, red) and UCP1 (green). ForAdipoTrak-GFPsuppression and reactivation studies,AdipoTrak-GFPmice were maintained on Dox from conception until 2 months of age (a,d,e). Dox was removed for 2 weeks and subsequently mice were maintained at RT or cold exposed for 7 days off Dox as shown ina. Subcutaneous inguinal adipose depot explants were imaged or sectioned and immunostained for reporter (GFP, false coloured red) and UCP1 (green) (e). Quantification of total UCP1+ beige adipocytes that were RFP+ is indicated to the right of the images. Images are representative fromn=4 mice per group replicated twice. Scale bar, 10 μm (b,d,f,h,j,l). Scale bar, 100 μm (c,e,g,i,k,m). Figure 1: Cre drivers with high beige adipocyte labelling. ( a – m ) Two-month-old male Cre mice ( AdipoTrak-Cre and SM22-Cre ); R26R RFP mouse models ( b , c , f , g ) were maintained at RT (23 °C) or cold exposed (6 °C) for 7 days as shown in a . Subcutaneous inguinal adipose depot explants were imaged for direct RFP fluorescence or sectioned and immunostained for reporter (RFP, red) and UCP1 (green); co-expression (RFP+UCP1) is a yellow-gold hue. Cell nuclei were counterstained with DAPI (blue). Two-month-old male, inducible Cre mice ( NG2-Cre ERT2 ; SMA-Cre ERT2 and SMA-rtTA-TRE-Cre ); R26R RFP mice ( h – m ) were administered one dose of TM on 2 consecutive days or administered Dox 3 days before experimentation. Mice were maintained at RT or cold exposed for 7 days as shown in a . Subcutaneous inguinal adipose depot explants were imaged or were sectioned and immunostained for reporter (RFP, red) and UCP1 (green). For AdipoTrak-GFP suppression and reactivation studies, AdipoTrak-GFP mice were maintained on Dox from conception until 2 months of age ( a , d , e ). Dox was removed for 2 weeks and subsequently mice were maintained at RT or cold exposed for 7 days off Dox as shown in a . Subcutaneous inguinal adipose depot explants were imaged or sectioned and immunostained for reporter (GFP, false coloured red) and UCP1 (green) ( e ). Quantification of total UCP1+ beige adipocytes that were RFP+ is indicated to the right of the images. Images are representative from n =4 mice per group replicated twice. Scale bar, 10 μm ( b , d , f , h , j , l ). Scale bar, 100 μm ( c , e , g , i , k , m ). Full size image To attempt to probe the adipose mural compartment and existing white adipocytes, two candidates for beige origin, we examined AdipoTrak ; RFP ( PPARγ tTA ; TRE-Cre; Rosa26R RFP ) mice [13] , [14] , [27] , [28] . The AdipoTrak system marks the entire white adipose lineage including mural resident progenitors and white adipocytes. Consistent with reports [13] , [14] , [27] , [28] , AdipoTrak ; RFP marked the adipose-mural vasculature and apparently 100% of white unilocular adipocytes within the inguinal and perigonadal adipose depots, both in whole depot images and in histological sections at both cold temperature and RT ( Fig. 1b,c and Supplementary Fig. 1a,b ). In histological sections of cold-exposed AdipoTrak; RFP mice, 100% of UCP1 + multilocular beige adipocytes appeared RFP+ in inguinal and perigonadal depots ( Fig. 1c and Supplementary Fig. 1b ). To attempt to probe the mural compartment in a more restricted manner, we turned to AdipoTrak; GFP ( PPARγ tTA ; TRE-H2B-GFP ) mice in which the green fluorescent protein (GFP) is incorporated into the chromatin of proliferating cells such as the mural cells and not into postmitotic cells such as existing white adipocytes. Nevertheless, GFP will be detected in the nuclei of adipocytes if they differentiate from a GFP-marked mural source [13] , [27] . We treated AdipoTrak; GFP mice with Dox, to suppress the tTA system, from conception until they reached 2 months of age. We then removed Dox for 2 weeks, to activate H2B-GFP in the proliferative mural progenitor cell pool and the few white adipocytes predicted to evolve from them during this time frame ( Fig. 1a , lower left illustration). Consistent with that notion, in RT-housed mice some perivascular mural cells were GFP labelled and <2% of adipocytes were GFP+ ( Fig. 1d,e ; the black deficit present within inguinal depots is a lymph node). However, when these mice were exposed to the cold we observed that GFP+ nuclei were no longer restricted at the vasculature and now marked a much greater fraction of the adipocyte compartment, as seen in whole depot images ( Fig. 1d , GFP is false coloured red in this image, to mirror the RFP colouring in Fig. 1b,f,h,j,i ). IHC analyses showed that ∼ 30%±10 of UCP1 + beige adipocytes were GFP+, suggesting that some beige adipocytes emanated from this AdipoTrak GFP + mural progenitor pool, which is only a subset of AdipoTrak + mural cells, those that proliferated in the brief Dox-off window ( Fig. 1e ). To further explore a possible mural source for beige adipocyte formation, we developed a series of mural cell Cre/inducible Cre; Rosa26R RFP mouse marking strains: SM22-Cre , NG2-Cre ERT2 , SMA-Cre ERT2 and SMA-rtTA; TRE-Cre [21] , [29] , [30] . We found that SM22 - (transgelin), NG2 - (chondroitin sulfate proteoglycan 4) and SMA -driven reporters marked vascular-resident mural cells in many tissues including adipose depots ( Fig. 1f–m and Supplementary Fig. 1c–j ), consistent with previous reports [3] , [21] , [31] , [32] , [33] . For example, SM22-Cre ; RFP marked the adipose tissue (subcutaneous and visceral) vasculature at RT in whole depot and IHC images ( Fig. 1f,g and Supplementary Fig. 1c,d ). This pattern elaborated on cold exposure with expansion of RFP expression in whole depots and in histology with 69%±19 of inguinal and 63%±13 of perigonadal UCP1 + beige adipocytes co-expressing RFP ( Fig. 1g and Supplementary Fig. 1d ). We also observed this pattern with two inducible mural cell Cre ( NG2-Cre ERT2 and SMA-Cre ERT2 ) mice that we randomized to either vehicle or to one dose of TM (250 mg kg −1 per day) for 2 consecutive days. Forty-eight hours after the last injection, we housed the mice for 7 days either at RT (23 °C) or in the cold (6 °C; Fig. 1a ). We found that NG2-Cre ERT2 ; RFP marked some mural cells and essentially 100% of adipocytes in subcutaneous adipose depots (inguinal and periscapular; Fig. 1h,i ). However, in visceral depots RFP marked only the mural vasculature and not adipocytes, providing a potential tool for the visceral location ( Supplementary Fig. 1e,f ). In response to the cold we observed that ∼ 51%±16 of subcutaneous inguinal and 49%±11 of visceral perigonadal UCP1 + beige adipocytes were RFP+ ( Fig. 1i and Supplementary Fig. 1f ). The fact that ∼ 100% of subcutaneous white adipocytes were labelled at RT and only ∼ 50% of UCP1 + beige cells were marked after cold exposure indicates that beige sources other than white adipocytes probably exist, the data supported by the results with the visceral beige marking outcomes. We next assessed SMA-Cre ERT2 ; RFP mice. At RT, RFP+ cells were present in mural vascular positions of all adipose depots but not in adipocytes of any adipose depot ( Fig. 1j,k and Supplementary Fig. 1g,h , not shown). On cold stimulation, RFP expression elaborated and we found that 60%±18 of subcutaneous inguinal and 65%±15 of visceral perigonadal UCP1 + beige adipocytes were RFP+ ( Fig. 1k and Supplementary Fig. 1g,h ). We observed similar results with a SMA-rtTA; RFP Dox-inducible mouse strain ( SMA-rtTA; TRE-Cre; Rosa26R RFP ). Dox was administered 3 days before 7 days of RT or cold exposure ( Fig. 1a ). At RT, RFP was restricted to the mural vasculature compartment in subcutaneous and visceral depots ( Fig. 1l,m and Supplementary Fig. 1i,j ). In response to the cold, SMA-rtTA; RFP marked the adipocyte compartment in whole depots, and in histology the RFP reporter fate mapped into 68%±15 and 55%±19 of UCP1 + beige adipocytes in the inguinal and perigonadal adipose depots, respectively ( Fig. 1l,m and Supplementary Fig. 1i,j ). Cre models with low beige-adipocyte labelling As the muscle has been proposed as a brown adipocyte source [9] , [34] , we tested two proposed muscle ( Myf5-Cre and Myogenin-Cre ) Cre strains. Myf5-Cre is reported to mark the muscle, classical interscapular brown adipose tissue (BAT), a subset of white adipose depots and a range of other tissues [9] , [18] , [34] . Myogenin-Cre is reported to mark the skeletal muscle lineage [35] . We found that Myf5-Cre; RFP fluorescence was absent in both the subcutaneous inguinal and the visceral perigonadal adipose depots at RT and after cold exposure, consistent with previous reports [9] ( Fig. 2a,b and Supplementary Fig. 2a,b ). The tool did mark adipocytes in other depots (please see below). For Myogenin-Cre ; RFP mice, we did not detect RFP fluorescence in any adipose depot at either temperature ( Fig. 2c,d and Supplementary Fig. 2c,d ). These data are consistent with the notion that lineages marked by Myf5-Cre and Myogenin-Cre are not sources of beige adipocytes in either inguinal (a major location of beige cells) or perigonadal depots, and in the case of the skeletal muscle Myogenin-Cre marking strain does not appear to be sources in any of the evaluated depots. 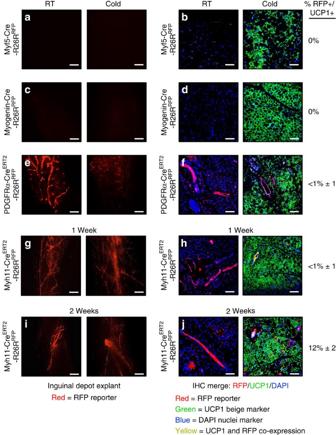Figure 2: Cre models with low beige adipocyte labelling. (a–h) Two-month-old male Cre mice (Myf5-CreandMyogenin (MyoG)-Cre);R26RRFPmouse models were maintained at RT (23 °C) or cold exposed (6 °C) for 7 days. Subcutaneous inguinal adipose depot explants were imaged for direct RFP fluorescence or sectioned and immunostained for reporter (RFP, red) and UCP1 (green) (a–d). Two-month-old male, inducible Cre mice (PDGFRα-CreERT2andMyh11-CreERT2);R26RRFPmice were administered one dose of TM on 2 consecutive days. Mice were maintained at RT or cold exposed for 7 days. Subcutaneous inguinal adipose depot explants were imaged or sectioned and immunostained for reporter (RFP, red) and UCP1 (green) (e–h). (i,j)Myh11-CreERT2; R26RRFPwere also housed in the cold or RT for 14 days. Subcutaneous inguinal adipose depot explants were imaged or sectioned and immunostained for reporter (RFP, red) and UCP1 (green). Quantification of UCP1+ beige adipocytes that were RFP+ is denoted next to the IHC image. Images are representative fromn=4 mice per group replicated twice. Scale bar, 10 μm (a,c,e,g,i). Scale bar, 100 μm (b,d,f,h,j). Figure 2: Cre models with low beige adipocyte labelling. ( a – h ) Two-month-old male Cre mice ( Myf5-Cre and Myogenin (MyoG)-Cre ); R26R RFP mouse models were maintained at RT (23 °C) or cold exposed (6 °C) for 7 days. Subcutaneous inguinal adipose depot explants were imaged for direct RFP fluorescence or sectioned and immunostained for reporter (RFP, red) and UCP1 (green) ( a – d ). Two-month-old male, inducible Cre mice ( PDGFRα-Cre ERT2 and Myh11-Cre ERT2 ); R26R RFP mice were administered one dose of TM on 2 consecutive days. Mice were maintained at RT or cold exposed for 7 days. Subcutaneous inguinal adipose depot explants were imaged or sectioned and immunostained for reporter (RFP, red) and UCP1 (green) ( e – h ). ( i , j ) Myh11-Cre ERT2 ; R26R RFP were also housed in the cold or RT for 14 days. Subcutaneous inguinal adipose depot explants were imaged or sectioned and immunostained for reporter (RFP, red) and UCP1 (green). Quantification of UCP1+ beige adipocytes that were RFP+ is denoted next to the IHC image. Images are representative from n =4 mice per group replicated twice. Scale bar, 10 μm ( a , c , e , g , i ). Scale bar, 100 μm ( b , d , f , h , j ). Full size image We also tested two previously reported beige adipocyte marking inducible Cre mice ( PDGFRα-Cre ERT2 and Myh11-Cre ERT2 ) [11] , [12] . Both PDGFRα and Myh11 are reported to mark the vascular compartment of many tissues [32] , [36] , [37] . In adipose depots, PDGFRα marking is reported to be located in non-mural perivascular cells and to mark 45% of β3-adregeneric-induced perigonadal beige adipocytes [12] . Myh11 is a well-described smooth muscle marker and is reported to mark a subset (15%) of cold-induced beige inguinal adipocytes [11] , [32] . We first examined PDGFRα-Cre ERT2 ; RFP mice and found that within adipose depots RFP was principally restricted to non-mural perivasculature positions, as previously reported [12] , at RT ( Fig. 2e,f and Supplementary Fig. 2e,f ). After cold exposure, RFP labelled 0–1%±1 of UCP1 + beige adipocytes and the few we could detect were scattered throughout the subcutaneous and visceral adipose depots ( Fig. 2f and Supplementary Fig. 2f ). Myh11-Cre ERT2 ; RFP marked the mural vascular compartment of all adipose depots at either cold temperature or RT ( Fig. 2g–j and Supplementary Fig. 2g–j ). After 7 days of cold exposure RFP labelled <1% of UCP1 + beige adipocytes but after 14 days of cold conditions ∼ 12%±2 and 10%±2 of inguinal and perigonadal UCP1 + beige adipocytes were RFP+, respectively, consistent with a previous report [11] ( Fig. 2i,j and Supplementary Fig. 2i,j ). Taken together, our data suggest that beige adipocytes are not primarily from an adipocyte, a myogenic or a PDGFRα source, but rather from a vascular-residing mural cell source, and that mice harbouring SMA-based genetically engineered tools might be useful strains to mark and track the beige lineage. White adipocytes do not generate cold-induced beige adipocytes To begin to probe the adipocyte compartment in a more restricted manner, we turned to two adipocyte-marking strains, adiponectin-Cre ERT2 and aP2-Cre ERT2 , and combined them with a Rosa26R RFP reporter allele. We administered one dose of TM for 2 consecutive days to 2-month-old male mice. Mice were maintained at RT for 1 week and then randomized them to 1 week of either RT or cold temperature. Of note, as RT is lower than thermo-neutrality, it can stimulate beige adipocyte formation [38] , [39] ( Fig. 3a ). We found that 2 days after TM administration, ‘pulse’, both drivers labelled essentially all adipocytes ( ∼ 99%±5; Fig. 3b,c and Supplementary Fig. 3a,b ). This included labelling of virtually all beige adipocytes that were present at RT (sub-thermo-neutral) conditions and before cold exposure ( Fig. 3b,c ). After cold stimulation, we found that the percentage of adipocyte driver-marked beige adipocytes dropped significantly to <40%. That is, the majority (60–70%±15) of cold-induced UCP1 + beige adipocytes appeared unlabelled (RFP negative) and to derive from a non-adipocyte source (white or existing beige). These percentages correspond quite closely to the percentage of beige cells labelled in the SMA-Cre ERT2 ; RFP or SMA-rtTA; RFP cold-induced fate-mapping studies ( Fig. 1j–m ). We also examined areas of the white depots that only contained white adipocytes, areas that lacked beige cells, for the possible presence of UCP1 expression. We found that in both adiponectin-Cre ERT2 ; RFP and aP2-Cre ERT2 ; RFP mouse models, unilocular white adipocytes did not express UCP1 ( Supplementary Fig. 3a,b ). The various amounts of adipocyte-driver-labelled (30–40%) and -unlabelled (60–70%) beige adipocytes, which do express adiponectin and aP2 (ref. 8 ), present after cold exposure. This could be reconciled by the existence of UCP1 + beige cells present at RT, as ambient temperatures are below thermo-neutrality and therefore are a beiging stimulus. To further explore the pre-existing beige adipocytes and the newly formed cold-induced beige cells, we turned to an UCP1-Cre ERT2 mouse strain and combined the driver with the Rosa26R RFP reporter allele. UCP1 is expressed in beige adipocytes but not in white adipocytes; thus, the eponymous driver strain can differentiate between beige adipocytes that are pre-existing, and marked by the UCP1 -driver, and perdure from white adipocytes, not labelled by the UCP1 driver, which could undergo a cold-induced transformation into beige cells. To attempt to discriminate between beige pre-existing and white transformation, we administered one dose of TM for 2 consecutive days to UCP1-Cre ERT2 ; RFP P60 male mice ( Fig. 3d ). Mice were maintained at RT and analysed at pulse (2 days post TM induction) to visualize and score existing beige adipocytes, and to determine the recombination efficiency of the reporter compared with endogenous UCP1 expression. We found, as reported [24] , [40] , [41] , that UCP1 + beige adipocytes existed in the P60 RT-housed mice, and that 90% of these UCP1 + beige adipocytes were RFP+, indicating a high correspondence between UCP1-Cre ERT2 -driven reporter marking and endogenous UCP1 expression/beige adipocytes ( Fig. 3d ). To attempt to estimate the percentages of beige adipocytes that perdure and those that form de novo after cold exposure, we TM activated the UCP1-Cre ERT2 ; RFP reporter to mark pre-existing beige adipocytes, waited a week and then randomized the mice to 7 days of RT or cold temperature ( Fig. 3d ). At RT, ∼ 90% of UCP1 + cells co-expressed the RFP reporter, just as at pulse, and cold exposure significantly reduced this to only ∼ 30% co-expression ( Fig. 3d ). This reduction from 90 to 30% roughly correlates to our fate-mapping results (60–70% marking) in which we studied cold-exposed SMA-Cre ERT2 ; RFP and SMA-rtTA; RFP mice. 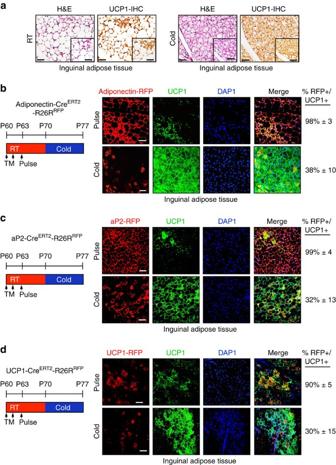Figure 3: Existing white adipocytes do not contribute to beiging. (a) Two-month old C57BL/6J mice were maintained at RT or cold temperature for 7 days. Subcutaneous inguinal adipose depots were haematoxylin and eosin (H&E) stained and IHC stained for UCP1. Insets are magnified images. Scale bar, 100 μm (in both images). (b–d) Two-month-oldAdiponectin-CreERT2; RFP(b),aP2-CreERT2: RFP(c) orUCP1-CreERT2; RFP(d) male mice were administered one dose of TM for 2 consecutive days and examined (pulse) or mice were maintained at RT for 7 days (TM washout period). Subsequently, mice were cold exposed for 7 days. Subcutaneous inguinal adipose depots were sectioned and immunostained for RFP (red) and UCP1 (green). Cell nuclei were visualized by DAPI staining. Quantification of UCP1+ beige adipocytes that were RFP+ is denoted next to the IHC image. Images are representative fromn=3 mice per group replicated twice. Scale bar, 100 μm. Figure 3: Existing white adipocytes do not contribute to beiging. ( a ) Two-month old C57BL/6J mice were maintained at RT or cold temperature for 7 days. Subcutaneous inguinal adipose depots were haematoxylin and eosin (H&E) stained and IHC stained for UCP1. Insets are magnified images. Scale bar, 100 μm (in both images). ( b – d ) Two-month-old Adiponectin-Cre ERT2 ; RFP ( b ), aP2-Cre ERT2 : RFP ( c ) or UCP1-Cre ERT2 ; RFP ( d ) male mice were administered one dose of TM for 2 consecutive days and examined (pulse) or mice were maintained at RT for 7 days (TM washout period). Subsequently, mice were cold exposed for 7 days. Subcutaneous inguinal adipose depots were sectioned and immunostained for RFP (red) and UCP1 (green). Cell nuclei were visualized by DAPI staining. Quantification of UCP1+ beige adipocytes that were RFP+ is denoted next to the IHC image. Images are representative from n =3 mice per group replicated twice. Scale bar, 100 μm. Full size image AdipoTrak and Myf5-Cre characterization AdipoTrak and Mfy5-Cre have been exploited to examine white and brown cell biology, and here we further examined the marking potential of these mouse strains in various adipose depots and organs [9] , [13] , [27] , [28] , [34] . To further examine AdipoTrak , we incorporated both a TRE-H2B-GFP reporter and a Rosa26R RFP reporter to generate a double reporter strain ( PPARγ tTA ; TRE-Cre; TRE-H2B-GFP; Rosa26R RFP ). We combined the two marking alleles, as they provide different information: TRE-H2B-GFP will report active AdipoTrak expression and Rosa26R RFP will report both active and historic AdipoTrak expression [13] . In this combined setting, yellow indicates both active and historic expression, whereas red indicates only historic AdipoTrak ( PPARγ ) expression in the absence of active expression ( Supplementary Fig. 4a ). We examined 2-month-old AdipoTrak; RFP; GFP mice and found that yellow (overlap between RFP and GFP) was only apparent in the adipose tissues ( Fig. 4a ). The brain, muscle and pancreas were RFP+ and lacked GFP expression, indicating that these tissues had AdipoTrak histories, consistent with our reports of embryonic AdipoTrak expression patterns [14] ( Fig. 4a ). These data, along with those in Fig. 1 , indicate that in adults AdipoTrak is principally restricted to adipose depots and may provide a tool to mark the beige progenitors and to fate map cold-induced beiging. 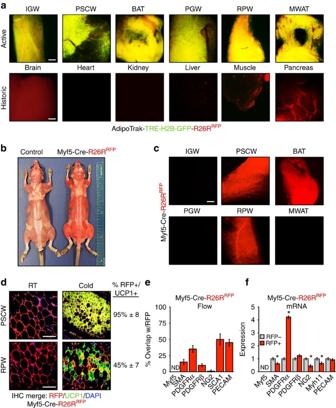Figure 4: AdipoTrak and Myf5 model characterization. (a) Merged (H2B-GFPand RFP) whole-mount images of denoted adipose depots and other tissues from 2-month-oldAdipoTrak (PPARγτTA,TRE-Cre); TRE-H2B-GFP; R26RRFPmale mice and control (PPARγtTA; RFP) mice. BAT, classical brown adipose tissue; IGW, inguinal; MWAT, mesenteric white adipose tissue; PGW, perigonadal; PSCW, periscapular; RPW, retroperitoneal. Scale bar, 10 μm. (b) Image of control (R26RRFP) andMyf5-Cre; RFPmale mice. Please note the RFP fluorescence was easily observed in regular room lighting from theMyf5-Cre; RFPmouse. (c) Fluorescence microscopic whole-mount images of RFP fluorescence from denoted adipose depots from 2-month-oldMyf5-Cre; RFPRT mice. Scale bar, 10 μm. (d) Two-month-oldMyf5-Cre; RFPmale mice were maintained at RT or cold exposed for 7 days. Histological sections from periscapular (top: PSCW) and retroperitoneal (bottom: RPW) adipose depots were examined for RFP fluorescence andUCP1(green) expression. Cell nuclei were counterstained with DAPI (blue). Quantification of UCP1+ beige adipocytes that were RFP+ is denoted next to the IHC image. (e) Adipose depot cells from 2-month-oldMyf5-Cre; RFPmice were analysed by flow cytometry for co-expression of RFP with the indicated genes. (f) Adipose depot cells from 2-month-oldMyf5-Cre; RFPmale mice were separated into RFP+ and RFP− fractions using FACS and examined for mRNA expression of denoted genes using qPCR. ND, not detected. Data are means±s.e.m. (n=4–5 mice per group replicated twice). Scale bar, 100 μm. Student’st-test, *P<0.05, RFP+ compared with RFP−. Figure 4: AdipoTrak and Myf5 model characterization. ( a ) Merged ( H2B-GFP and RFP) whole-mount images of denoted adipose depots and other tissues from 2-month-old AdipoTrak (PPARγ τTA ,TRE-Cre); TRE-H2B-GFP; R26R RFP male mice and control ( PPARγ tTA ; RFP ) mice. BAT, classical brown adipose tissue; IGW, inguinal; MWAT, mesenteric white adipose tissue; PGW, perigonadal; PSCW, periscapular; RPW, retroperitoneal. Scale bar, 10 μm. ( b ) Image of control ( R26R RFP ) and Myf5-Cre; RFP male mice. Please note the RFP fluorescence was easily observed in regular room lighting from the Myf5-Cre; RFP mouse. ( c ) Fluorescence microscopic whole-mount images of RFP fluorescence from denoted adipose depots from 2-month-old Myf5-Cre; RFP RT mice. Scale bar, 10 μm. ( d ) Two-month-old Myf5-Cre; RFP male mice were maintained at RT or cold exposed for 7 days. Histological sections from periscapular (top: PSCW) and retroperitoneal (bottom: RPW) adipose depots were examined for RFP fluorescence and UCP1 (green) expression. Cell nuclei were counterstained with DAPI (blue). Quantification of UCP1+ beige adipocytes that were RFP+ is denoted next to the IHC image. ( e ) Adipose depot cells from 2-month-old Myf5-Cre; RFP mice were analysed by flow cytometry for co-expression of RFP with the indicated genes. ( f ) Adipose depot cells from 2-month-old Myf5-Cre; RFP male mice were separated into RFP+ and RFP− fractions using FACS and examined for mRNA expression of denoted genes using qPCR. ND, not detected. Data are means±s.e.m. ( n =4–5 mice per group replicated twice). Scale bar, 100 μm. Student’s t -test, * P <0.05, RFP+ compared with RFP−. Full size image We next examined Myf5-Cre mice [42] for RFP expression in day 17.5 embryos (E17.5) and in 2-month-old adult mice ( Supplementary Fig. 4b ). We found that Myf5-Cre E17.5 embryos and 2-month-old mice were visibly red, that is, even in the absence of fluorescent microscopy, indicative of robust fluorescence ( Fig. 4b and Supplementary Fig. 4c , left panel). Fluorescence imaging of embryos showed that the dorsal region, craniofacial region, front and hind limbs, and the tail were RFP+, and the liver and the eyes were the only tissues in which we did not detect RFP ( Supplementary Fig. 4c , right panel). This broad RFP expression was also observed in 2-month-old Myf5-Cre mice. RFP was detected in the brain, classical BAT, kidney, liver, lymph nodes, skeletal muscle, pancreas and skin ( Supplementary Fig. 4d ). Consistent with reports [9] , [34] , [43] , Myf5-Cre; RFP did not mark inguinal, perigonadal or mesenteric white adipose depots but did mark periscapular and retroperitoneal white adipose tissue and essentially all unilocular white adipocytes in these two depots appeared RFP+ ( Fig. 4c,d ). In the periscapular and retroperitoneal adipose depots, Myf5-Cre; RFP marking seemed quite indiscriminate, labelling what appeared to be essentially every cell type. For example, in adipose vessels, Myf5-Cre; RFP marked the endothelial cells, mural cells and other perivascular cells ( Supplementary Fig. 4e , not shown). The widespread expression observed in histology was supported by flow cytometric analyses. For example, ∼ 55% of all stromal vascular fraction (SVF) cells were RFP+ ( Supplementary Fig. 4f ) and these cells encompassed mural lineages, endothelial lineages, immune cells, PDGFRα cells and so on. Quantitative PCR (qPCR) studies examining fluorescence-activated cell sorting (FACS)-isolated RFP− and RFP+ cells indicated that Myf5/RFP + cells were not enriched in adipocyte progenitor, mural and endothelial cell markers, and in large part the RFP− and RFP+ cells had similar expression patterns ( Fig. 4f ). We also attempted to test whether the RFP expression in the adipose depots reflected active or historic Myf5 expression by using both flow cytometric analyses of RFP+ cells and qPCR analyses of FACS-isolated RFP+ cells. Based on these studies the RFP+ cells did not appear to express Myf5 protein or messenger RNA ( Fig. 4e,f ); that is, the RFP expression was based on historic Cre activity. We next examined whether the historic Myf5-Cre -driven RFP expression would mark cold-induced beige cells. Histological studies from Myf5-Cre; RFP mice housed in the cold showed that 95% of periscapular and 45% of retroperitoneal UCP1 + beige adipocytes were RFP+ ( Fig. 4d ). Taken together, the remarkably general marking, lack of inducibility and non-correspondence of endogenous expression to Cre-driven marking appear to be significant issues for the Myf5 stain in adipose biology and probably confound interpretation and utility. SMA-Cre ERT2 white adipocyte characterization Transdifferentiation of mature unilocular white adipocytes has been proposed as a source of beige adipocytes [5] , [6] . However, our data suggest that cells expressing a mural cell genetic signature ( SM22 +, Myh11 +, NG2 + and SMA +) are a key source of cold-induced beige adipocytes. A possible reconciliation of the observations that the smooth muscle/mural drivers fate map into beige cells with the theorized white adipocyte transdifferentiation is that mature white adipocytes could express mural markers or marking strain-driven RFP, similar to what we observed with NG2-Cre ERT2 and a subset of subcutaneous white adipocytes ( Fig. 1i ). To explore this possibility, we further characterized endogenous SMA expression and SMA-Cre ERT2 ; RFP expression ( Supplementary Fig. 5a ) in white adipose depots with a focus on potential expression in adipocytes. We evaluated endogenous SMA expression in depots of wild-type mice using IHC. In these studies, endogenous SMA appeared restricted to the adipose tissue vasculature in all depots (subcutaneous and visceral) and it did not appear to be expressed in any examined mature white adipocytes ( Fig. 5a,b ). We also assessed endogenous SMA expression and SMA-Cre ERT2 -driven RFP expression in SMA-Cre ERT2 ; RFP mice. In the uninduced (no TM) state, we again observed, by IHC, that endogenous SMA was restricted to the vasculature of all adipose depots (subcutaneous and visceral), and that endogenous SMA was not expressed in adipocytes ( Fig. 5c ). We also found that RFP fluorescence was not induced in the absence of TM ( Fig. 5c ). We then examined SMA and RFP expression in the SMA-Cre ERT2 ; RFP setting 2 days after administering TM. We found that endogenous SMA and SMA-Cre ERT2 -driven RFP were restricted to the adipose tissue vasculature and were not expressed in adipocytes ( Fig. 5d ). 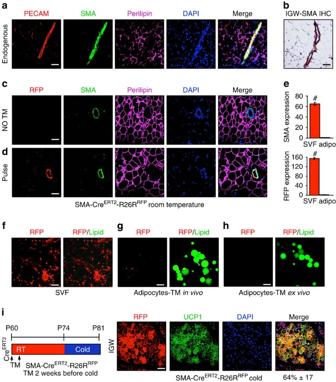Figure 5: SMA-CreERT2characterization. (a) Subcutaneous inguinal adipose depots from RT 2-month-old wild-type male mice were immunostained forPECAM,SMAandperilipin, and nuclei detected with DAPI. (b) Subcutaneous inguinal adipose depots from RT 2-month-old wild-type male mice were IHC stained for endogenous SMA. (c) Subcutaneous inguinal adipose depots from 2-month-old uninduced (no TM)SMA-CreERT2; RFPmale mice were immunostained for RFP, SMA and perilipin, and nuclei stained with DAPI. (d) Subcutaneous inguinal adipose depot from 2-month-old pulsedSMA-CreERT2; RFPmale mice were immunostained for RFP,SMAandperilipin, and nuclei highlighted with DAPI. (e) SV cells and adipocytes were isolated from 2-month-old TM-pulsedSMA-CreERT2; RFPmale mice and mRNA expression of endogenousSMAand SMA-driven RFP were assessed by qPCR. Data are means±s.e.m. (n=4–5 mice per group replicated thrice). Student’st-test, #P<0.001, SVF compared with adipocyte compartment. (f) SV cells were isolated from 2-month-old TM-pulsedSMA-CreERT2; RFPmale mice and visualized for RFP and lipid (green; LipidTox green). (g) Adipocytes were floatation isolated from 2-month-old TM-pulsed inducedSMA-CreERT2; RFPmale mice and visualized for RFP and lipid (green). (h) Adipocytes were isolated from 2-month-old uninducedSMA-CreERT2; RFPmale mice. TM was then administeredex vivofor 24 h and the floated adipocytes examined for RFP and lipid (green). (i) Two-month-oldSMA-CreERT2; RFPmale mice were administered one dose of TM for 2 consecutive days. Mice were maintained at RT for 14 days (TM washout). Mice were subsequently cold exposed for 7 days. Subcutaneous inguinal adipose depots were immunostained for RFP (red) andUCP1(green). Cell nuclei were counterstained with DAPI (blue). Quantification ofUCP1+ beige adipocytes that were RFP+ is denoted next to the IHC image. Images are representative fromn=4 mice per group replicated twice. Scale bar, 100 μm. Figure 5: SMA-Cre ERT2 characterization. ( a ) Subcutaneous inguinal adipose depots from RT 2-month-old wild-type male mice were immunostained for PECAM , SMA and perilipin , and nuclei detected with DAPI. ( b ) Subcutaneous inguinal adipose depots from RT 2-month-old wild-type male mice were IHC stained for endogenous SMA. ( c ) Subcutaneous inguinal adipose depots from 2-month-old uninduced (no TM) SMA-Cre ERT2 ; RFP male mice were immunostained for RFP, SMA and perilipin, and nuclei stained with DAPI. ( d ) Subcutaneous inguinal adipose depot from 2-month-old pulsed SMA-Cre ERT2 ; RFP male mice were immunostained for RFP, SMA and perilipin , and nuclei highlighted with DAPI. ( e ) SV cells and adipocytes were isolated from 2-month-old TM-pulsed SMA-Cre ERT2 ; RFP male mice and mRNA expression of endogenous SMA and SMA-driven RFP were assessed by qPCR. Data are means±s.e.m. ( n =4–5 mice per group replicated thrice). Student’s t -test, # P <0.001, SVF compared with adipocyte compartment. ( f ) SV cells were isolated from 2-month-old TM-pulsed SMA-Cre ERT2 ; RFP male mice and visualized for RFP and lipid (green; LipidTox green). ( g ) Adipocytes were floatation isolated from 2-month-old TM-pulsed induced SMA-Cre ERT2 ; RFP male mice and visualized for RFP and lipid (green). ( h ) Adipocytes were isolated from 2-month-old uninduced SMA-Cre ERT2 ; RFP male mice. TM was then administered ex vivo for 24 h and the floated adipocytes examined for RFP and lipid (green). ( i ) Two-month-old SMA-Cre ERT2 ; RFP male mice were administered one dose of TM for 2 consecutive days. Mice were maintained at RT for 14 days (TM washout). Mice were subsequently cold exposed for 7 days. Subcutaneous inguinal adipose depots were immunostained for RFP (red) and UCP1 (green). Cell nuclei were counterstained with DAPI (blue). Quantification of UCP1 + beige adipocytes that were RFP+ is denoted next to the IHC image. Images are representative from n =4 mice per group replicated twice. Scale bar, 100 μm. Full size image To further examine the possibility that SMA is expressed in adipocytes, we isolated both stromal vascular (SV) cells and floated adipocytes from RT-housed SMA-Cre ERT2 ; RFP mice 2 days after administering TM. We then quantified endogenous SMA and SMA-Cre ERT2 -driven RFP mRNA expression with qPCR. We found that SMA and RFP mRNA appeared to be expressed only in the SV compartment and we did not detect appreciable signal in the adipocyte fraction ( Fig. 5e ). We next examined individual SV cells and individual adipocytes, scoring over 5,000, for RFP expression. For this, we also stained the SV cells and the floated adipocytes, and with LipidTox Green, to highlight lipids. In the fluorescent microscopic examinations, we did not detect any adipocytes that expressed RFP, unlike the positive control SV compartment ( Fig. 5f,g ). We performed an analogous series of studies, first isolating adipocytes and then administered TM to induce reporter expression ex vivo ( Fig. 5h ). Again, we obtained similar results: no RFP expression in adipocytes. We next turned to cell culture studies, to examine the dynamics of SMA expression during white and beige adipogenesis, and to further test whether SMA might be expressed in cell culture-induced mature white or beige adipocytes. For this, we isolated SV cells, which contained the SMA -positive mural compartment ( Fig. 5e ), and cultured them for 7 days in white or beige adipogenic conditions and quantified endogenous SMA expression. We found that on either adipogenic induction SMA expression was rapidly and sustainably reduced ( Supplementary Fig. 5c ). We also examined the possibility that TM may perdure beyond the 2-day interval after administration and activate SMA-Cre ERT2 in mature beige or white adipocytes during the cold exposure period. For this, we extended the washout period to 14 days, administering TM to SMA-Cre ERT2 ; RFP P60 mice, waiting 2 weeks before cold exposure and then examining P81 mice. We found that SMA -marked cells, after a longer TM washout period, still fate mapped into cold-induced beige adipocytes at roughly the same percentage as we previously observed with the 2-day interval (64%±17; Fig. 5i ). Endogenous SMA and SMA-Cre ERT2 -driven RFP, before cold exposure, appeared to be restricted to the mural vascular compartment in several studies including IHC. The IHC studies also indicated that RFP and endogenous SMA expression had high concordance ( Fig. 5d ). We further examined potential concordance of endogenous SMA and the RFP signal using flow cytometry, to determine whether RFP-positive cells faithfully co-expressed SMA using cells isolated from SMA-Cre ERT2 ; RFP mice 2 days after TM administration (pulse). We found that virtually all RFP+ cells were SMA +, based on antibody staining for SMA ( Supplementary Fig. 5d ). The RFP-positive cells constituted about 50% of the total SMA population ( Supplementary Fig. 5e ). We also characterized the RFP-positive cells in flow cytometry and qPCR studies, finding that the RFP+ cells were enriched in adipocyte progenitor and mural cell markers but not in endothelial cell markers ( Supplementary Fig. 5f,g ). We also examined classical BAT for endogenous SMA expression and for SMA-Cre ERT2 -driven RFP reporter expression. At RT or after cold exposure, both endogenous SMA and RFP were restricted to the vasculature and were not expressed in mature brown adipocytes ( Supplementary Fig. 5h,i ). SMA-rtTA white adipocyte characterization We next examined SMA-rtTA; RFP (SMA-rtTA; TRE-Cre; Rosa26R RFP ) mice ( Supplementary Fig. 6a ) using similar tests to those performed on the SMA-Cre ERT2 ; RFP mice. We first inspected SMA-rtTA; RFP mice in the uninduced (no Dox) state. We observed, by IHC, that endogenous SMA was restricted to the adipose tissue vasculature, that endogenous SMA was not present in adipocytes, and that RFP fluorescence was not expressed in the absence of Dox ( Fig. 6a ). We then examined the RFP expression pattern in adipose depots of SMA-rtTA; RFP mice 2 days after Dox administration (pulse). RFP was restricted to the adipose tissue vasculature and aligned with endogenous perivascular SMA , adjacent to PECAM , in all adipose depots. RFP was not visible in adipocytes ( Fig. 5b,d ). We also generated SV and floated adipocyte fractions from RT Dox-pulsed SMA-rtTA; RFP mice and quantified RFP expression with qPCR. RFP was abundantly expressed in SV cells but not in adipocytes ( Fig. 6c ). We also floated adipocytes after a Dox pulse and examined them for RFP expression and for lipid staining. We did not detect RFP fluorescence in any adipocytes ( Fig. 6e ); over 5,000 adipocytes were examined in each analysis. We next analysed RFP+ and RFP− cells with flow cytometry and found that ∼ 97% of RFP+ cells co-expressed SMA ( Fig. 6f ). qPCR evaluation of flow cytometry-sorted RFP+ and RFP− cells showed that endogenous SMA was enriched in the RFP+ cell fraction ( Fig. 6g ). We further examined RFP+ cells by flow cytometry and qPCR, and found that RFP+ cells were enriched in mural and adipose progenitor markers, while lacking expression of endothelial or adipocyte markers ( Fig. 6h,i , not shown). 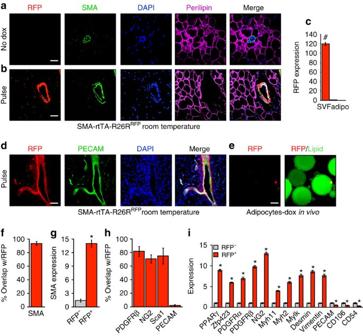Figure 6: SMA-rtTA characterization. (a) Subcutaneous inguinal adipose depots from 2-month old uninduced (no Dox)SMA-rtTA; RFP(SMA-rtTA; TRE-Cre; R26RRFP) male mice maintained at RT were immunostained for RFP, SMA and perilipin. Cell nuclei were counterstained with DAPI (blue). (b) Subcutaneous inguinal adipose depot sections from 2-month old Dox-pulseSMA-rtTA; RFPmale mice maintained at RT were immunostained for RFP, SMA and perilipin; nuclei were highlighted with DAPI. (c) SV cells and adipocytes were isolated from 2-month old pulseSMA-rtTA; RFPmale mice maintained at RT. mRNA expression of RFP were assessed by qPCR. Data are means±s.e.m. (n=4–5 mice per group). Studentst-test, #P-value <0.001, SVF compared with adipocyte compartment. (d) Subcutaneous inguinal adipose depots from 2-month old pulsedSMA-rtTA; RFPmale mice maintained at RT were sectioned and immunostained for RFP andPECAM(green), and nuclei stained with DAPI. (e) Adipocytes were isolated pulseSMA-rtTA; RFPmice described indand visualized for RFP and lipid (green). (f) Adipose depot cells of pulseSMA-rtTA; RFPmice as described indwere analysed for co-expression of RFP and SMA. (g) RFP− and RFP+ cells were FACS isolated from pulseSMA-rtTA; RFPmice andSMAmRNA expression was assessed using qPCR. (h) Adipose cells of pulseSMA-rtTA; RFPmice were flow analysed for co-expression of RFP with mural or endothelial markers. (i) RFP− and RFP+ cells were FACS isolated from pulseSMA-rtTA; RFPmice and mRNA expression of various adipose progenitor, mural and endothelial markers were assessed by qPCR. Data are means±s.e.m. (n=5 mice per group replicated twice). Images are representative fromn=4 mice per group replicated twice. Scale bar, 100 μm. Studentst-test, *P-value <0.01, RFP+ compared with RFP−. Figure 6: SMA-rtTA characterization. ( a ) Subcutaneous inguinal adipose depots from 2-month old uninduced (no Dox) SMA-rtTA; RFP ( SMA-rtTA; TRE-Cre; R26R RFP ) male mice maintained at RT were immunostained for RFP, SMA and perilipin. Cell nuclei were counterstained with DAPI (blue). ( b ) Subcutaneous inguinal adipose depot sections from 2-month old Dox-pulse SMA-rtTA; RFP male mice maintained at RT were immunostained for RFP, SMA and perilipin; nuclei were highlighted with DAPI. ( c ) SV cells and adipocytes were isolated from 2-month old pulse SMA-rtTA; RFP male mice maintained at RT. mRNA expression of RFP were assessed by qPCR. Data are means±s.e.m. ( n =4–5 mice per group). Students t -test, # P -value <0.001, SVF compared with adipocyte compartment. ( d ) Subcutaneous inguinal adipose depots from 2-month old pulsed SMA-rtTA; RFP male mice maintained at RT were sectioned and immunostained for RFP and PECAM (green), and nuclei stained with DAPI. ( e ) Adipocytes were isolated pulse SMA-rtTA; RFP mice described in d and visualized for RFP and lipid (green). ( f ) Adipose depot cells of pulse SMA-rtTA; RFP mice as described in d were analysed for co-expression of RFP and SMA. ( g ) RFP− and RFP+ cells were FACS isolated from pulse SMA-rtTA; RFP mice and SMA mRNA expression was assessed using qPCR. ( h ) Adipose cells of pulse SMA-rtTA; RFP mice were flow analysed for co-expression of RFP with mural or endothelial markers. ( i ) RFP− and RFP+ cells were FACS isolated from pulse SMA-rtTA; RFP mice and mRNA expression of various adipose progenitor, mural and endothelial markers were assessed by qPCR. Data are means±s.e.m. ( n =5 mice per group replicated twice). Images are representative from n =4 mice per group replicated twice. Scale bar, 100 μm. Students t -test, * P -value <0.01, RFP+ compared with RFP−. Full size image We then examined other tissues for SMA-Cre ERT2 - and SMA-rtTA -driven RFP expression. We found that both models had similar tissue expression patterns ( Supplementary Fig. 6b,c ). In both models, RFP labelled the vasculature and smooth muscle of the brain, cardiac and skeletal muscle (although to different levels), intestine, kidney, lung, the testes and the uterus ( Supplementary Fig. 6b,c , not shown). We also probed the SMA-rtTA -driven RFP reporter for expression in classical interscapular BAT. We found that the reporter was not expressed in mature brown adipocytes and remained at the vascular under both RT and cold conditions ( Supplementary Fig. 6d ). Together, the SMA-Cre ERT2 and SMA-rtTA experiments support the concordance of endogenous SMA , and SMA-Cre ERT2 - and SMA-rtTA -driven RFP expression. SMA characterization in beige adipocytes In the detailed characterizations described in Figs 5 and 6 and in Supplementary Figs 5 and 6 , endogenous SMA expression and SMA -driven reporter expression appeared restricted to the mural compartment, and expression was not observed in mature white adipocytes under RT conditions. During in vitro beige adipogenic induction of inguinal SV cells, SMA mRNA expression was rapidly reduced (within 24 h) and this suppressed expression was sustained throughout the remainder of beige adipocyte differentiation ( Supplementary Fig. 5c ). However, it could be possible that endogenous SMA is expressed in white and beige adipocytes on in vivo cold exposure. To assess this, we housed wild-type mice in the cold for 7 days. We then examined expression of endogenous SMA using immunofluorescence staining and found that after cold exposure endogenous SMA expression remained restricted to the vasculature and was not expressed in UCP1 + beige adipocytes or in UCP1 − white adipocytes ( Fig. 7a,b ). We continued to pursue the possibility that endogenous SMA might be expressed in white and/or beige adipocytes, by using two genetic strains to fluorescently highlight these two adipocyte cell types: Adiponectin-Cre ERT2 ; RFP (white and beige) and UCP1- Cre ERT2 ; RFP (beige). We housed uninduced (no TM) 2-month-old UCP1-Cre ERT2 ; RFP and Adiponectin-Cre ERT2 ; RFP male mice in the cold for 7 days, to stimulate de novo beige adipocyte formation. After cold exposure, we administered one dose of TM and maintained the mice at RT for 24 h ( Fig. 7c,d ). We found that UCP1-Cre ERT2 ; RFP marked ∼ 90%±7 of all UCP1 + immunostained beige adipocytes, indicating high correspondence between reporter and endogenous UCP1 expression. We did not detect, by immunostaining, endogenous SMA expression in any UCP1 -driven RFP-marked mature beige adipocytes. Rather, endogenous SMA remained restricted to the vascular compartment ( Fig. 7c ). We observed similar results with the Adiponectin-Cre ERT2 ; RFP strain. RFP labelled all (100%±6) white and beige adipocytes; however, endogenous SMA expression was restricted to the vessel and did not overlap with Adiponectin-Cre ERT2 ; RFP labelling ( Fig. 7d ). 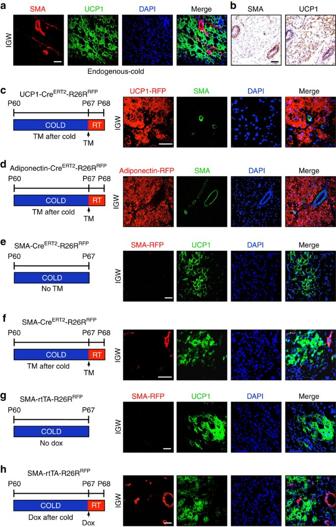Figure 7: Endogenous SMA and SMA-driven reporter expression profile in beige adipocytes. (a) Subcutaneous adipose depots from 2-month-old, cold-exposed wild-type mice were immunostained for endogenousSMAandUCP1expression, and nuclei detected with DAPI. (b) Subcutaneous adipose depots from 2-month-old, cold-exposed wild-type male mice were IHC stained for endogenous SMA andUCP1. (c,d) Two-month-old uninduced (no TM)UCP1-CreERT2(c) orAdiponectin-CreERT2(d) male mice were cold exposed. After 7 days of cold exposure, mice were administered TM and maintained at RT for 24 h. Subcutaneous inguinal adipose depots were immunostained for RFP and UCP1 (green); nuclei were highlighted with DAPI. (e) Subcutaneous adipose depots from cold-exposed uninducedSMA-CreERT2; RFPwere immunostained for RFP and UCP1 (green); nuclei were highlighted with DAPI. (f) UninducedSMA-CreERT2; RFPmice were cold exposed for 7 days; mice were then pulsed with TM and housed at RT for 24 h. Sections from the subcutaneous inguinal adipose depots were immunostained for RFP and UCP1 (green). Cell nuclei were counterstained with DAPI (blue). (g) UninducedSMA-rtTA; RFPmice were exposed to cold for 7 days. Subcutaneous inguinal adipose depot were sectioned and immunostained for RFP and UCP1 (green). Cell nuclei were counterstained with DAPI (blue). (h) UninducedSMA-rtTA; RFPmice were cold exposed for 7 days and then administered Dox for 24 h and maintained at RT. Subcutaneous inguinal adipose depot sections were analysed for RFP (red), UCP1 (green) and DAPI (blue). Figure 7: Endogenous SMA and SMA-driven reporter expression profile in beige adipocytes. ( a ) Subcutaneous adipose depots from 2-month-old, cold-exposed wild-type mice were immunostained for endogenous SMA and UCP1 expression, and nuclei detected with DAPI. ( b ) Subcutaneous adipose depots from 2-month-old, cold-exposed wild-type male mice were IHC stained for endogenous SMA and UCP1 . ( c , d ) Two-month-old uninduced (no TM) UCP1-Cre ERT2 ( c ) or Adiponectin-Cre ERT2 ( d ) male mice were cold exposed. After 7 days of cold exposure, mice were administered TM and maintained at RT for 24 h. Subcutaneous inguinal adipose depots were immunostained for RFP and UCP1 (green); nuclei were highlighted with DAPI. ( e ) Subcutaneous adipose depots from cold-exposed uninduced SMA-Cre ERT2 ; RFP were immunostained for RFP and UCP1 (green); nuclei were highlighted with DAPI. ( f ) Uninduced SMA-Cre ERT2 ; RFP mice were cold exposed for 7 days; mice were then pulsed with TM and housed at RT for 24 h. Sections from the subcutaneous inguinal adipose depots were immunostained for RFP and UCP1 (green). Cell nuclei were counterstained with DAPI (blue). ( g ) Uninduced SMA-rtTA; RFP mice were exposed to cold for 7 days. Subcutaneous inguinal adipose depot were sectioned and immunostained for RFP and UCP1 (green). Cell nuclei were counterstained with DAPI (blue). ( h ) Uninduced SMA-rtTA; RFP mice were cold exposed for 7 days and then administered Dox for 24 h and maintained at RT. Subcutaneous inguinal adipose depot sections were analysed for RFP (red), UCP1 (green) and DAPI (blue). Full size image We next used a similar series of tests to determine whether SMA -driven RFP expression might be induced in response to cold temperatures. For this, we examined RFP expression in cold-exposed SMA-Cre ERT2 ; RFP mice that had never been administered TM ( Fig. 7e,f ). In these uninduced cold-exposed specimens, we did not detect RFP fluorescence ( Fig. 7e ). We next housed 2-month old uninduced SMA-Cre ERT2 ; RFP male mice in the cold and after a week we induced reporter expression with a dose of TM. When induced after the cold, RFP expression appeared restricted to the blood vessels and we did not detect RFP expression in UCP1 + beige adipocytes ( Fig. 7f ). We next repeated these studies using cold-exposed SMA-rtTA; RFP mice that were never administered Dox or were administered Dox after a week of cold ( Fig. 7g,h ). In the uninduced (no Dox) specimens, we did not detect RFP fluorescence ( Fig. 7g ). When the mice received Dox induction after cold exposure, RFP fluorescence appeared restricted to the vasculature and was not detected in UCP1 + beige adipocytes ( Fig. 7h ). The various approaches and methods indicate that endogenous SMA , SMA-Cre ERT2 -driven RFP and SMA-rtTA- driven RFP are not expressed in white or beige adipocytes. Rather, they appear to be present in the vascular compartment, although RFP does fate map into de novo beige adipocytes on cold exposure. SMA and Myh11 mark different mural cell compartments The SM22-Cre driver, both SMA drivers and the Myh11-Cre ERT2 driver marked the perivascular compartment and, in a restricted manner, with no apparent marking of adipocytes ( Figs 1 and 2 and Supplementary Figs 1 and 2 ). All four of these marking strains marked cold-induced beige cells, albeit with different frequencies: SM22 and the two inducible SMA drivers did so at a similarly high percentage (60–70%), whereas the inducible Myh11 driver did so at a low percentage ( Figs 1 and 2 and Supplementary Figs 1 and 2 ). This discrepancy could be accounted for if the various marking strains drive RFP expression in different cell types. To assess this notion, we immunostained histological samples derived from P60 SM22-Cre; RFP adipose depots with antibodies directed against SMA and Myh11 . We found a fairly high concordance of expression of endogenous SMA with SM22 -RFP. However, endogenous Myh11 staining overlapped with SM22 -RFP less frequently ( Supplementary Fig. 7a,b ). Flow cytometric studies, using antibodies directed against SMA , NG2 , Myh11 and PECAM endothelial marker, also indicated a diversity of marking: ∼ 55% of SM22-RFP cells co-expressed SMA , ∼ 40% of SM22-RFP cells co-expressed Myh11 and ∼ 15% of SM22-RFP cells co-expressed NG2 ; co-expression with PECAM was minimal ( Supplementary Fig. 7c ). We also FACS-isolated SM22-RFP+ and SM22-RFP − cells and quantified the levels of expression in the isolated cells for expression of SMA and Myh11 , of other mural cell markers and of endothelial markers. We found that SM22 and SMA were quite enriched in the SM22-RFP + cells, and that although Myh11 levels were higher in the SM22-RFP + compared with SM22-RFP − cells, the enrichment was to a lesser extent ( Supplementary Fig. 7d ). NG2 had roughly equal expression in SM22-RFP + and SM22-RFP − cells, PDGFRβ enrichment was closer to the SMA patterns and PECAM expression was higher in the SM22-RFP − cells. We next examined and compared inguinal adipose depots for endogenous expression of Myh11 and SMA . We found that Myh11 and SMA expression overlapped on some vessels, whereas in other vessels there was no co-expression ( Supplementary Fig. 7e ). This heterogeneous pattern was recapitulated in TM-pulsed Myh11-Cre ERT2 ; RFP mice, in comparisons of RFP and endogenous SMA expression. We found that Myh11-RFP + cells marked the vasculature of the inguinal adipose depots, and that only some vessels showed co-localization of Myh11-RFP and SMA ( Supplementary Fig. 7f ). We also flow cytometrically profiled the Myh11-Cre ERT2 ; RFP cells. We found that ∼ 98% of Myh11-RFP + cells co-expressed endogenous Myh11 , and that about ∼ 60% of the total number of immunostained Myh11 cells expressed Myh11-Cre ERT2 -driven RFP ( Supplementary Fig. 7g,h ). The flow cytometry studies also supported the diversity of Myh11 , SMA expression: ∼ 35% of the Myh11-RFP cells co-expressed Myh11 and ∼ 60% of Myh11-RFP cells immunostained with SMA , whereas only ∼ 25% of the antibody-positive SMA cells co-expressed RFP ( Supplementary Fig. 7i,j ). We also examined the expression levels of the various mural markers in FACS-isolated Myh11-Cre ERT2 ; RFP + and RFP− cells. We found that Myh11 was highly enriched in the Myh11-RFP + cells; both SMA and NG2 were enriched, but to a lesser extent ( Supplementary Fig. 7i,k ). Together, the IHC, flow cytometry and qPCR studies indicate that there is only partial overlap between several mural cell markers, and that, similar to what is observed in other tissues and organs [21] , [29] , [30] , [31] , [42] , there is a significant mural cell and vascular cell heterogeneity within adipose depots, potentially accounting for the different percentage of fate-mapping results we observed with the different mural cell-driver mouse strains. Elucidation of the biological basis of this heterogeneity may help clarify why the inducible SMA -driven tools appear to have the best characteristics for analysing beige biology. SMA-Cre ERT2 -expressing cells are necessary for beiging To test potential necessity of SMA-Cre ERT2 -expressing cells for cold-induced beiging, we attempted two strategies as follows: (1) a cell-killing strategy (diphtheria toxin fragment A ( DTA )) [44] and (2) a blockade of adipocyte differentiation ( PPARγ deletion) [45] , [46] . The PPARγ conditional deletion experiments were designed to test the requirement of SMA mural cells to generate beige adipocytes, by blocking their ability to differentiate, not the essential role of PPARγ in adipogenesis [47] . A concern of these approaches is that the SMA tools are expressed in mural compartments of many tissues and organs, and also mark other muscle types ( Supplementary Fig. 6c,d ) [21] . In addition, it also seems likely to be that even in adipose depots SMA is expressed in many mural cells that do not possess progenitor potential. Thus, non-autonomous issues may cloud the data, as many cellular debris created by the DTA cell-killing strategy. To attempt to minimize some of these concerns, the studies were conducted in a temporally regulated manner and proximate to cold exposure ( Supplementary Fig. 8a ). For these studies, we integrated conditional Rosa26R-DTA or conditional PPARγ fl/fl alleles with the inducible SMA-Cre ERT2 driver strain. We then randomized SMA-DTA and SMA-PPARγ fl/fl mice to vehicle or TM and to RT or cold temperature ( Supplementary Fig. 8a ). Vehicle-treated mice and mice lacking a salient allele (for example, no DTA ) served as negative controls. Both strategies ( DTA and PPARγ fl/fl ) appeared to inhibit cold-induced beige adipocyte formation and appeared to alter the physiological responses to cold exposure ( Fig. 8a–e ). For example, the induced SMA-DTA and SMA-PPARγ fl/fl mice had reduced body temperatures, elevated blood glucose levels, significant reductions in the quantities of multilocular or UCP1 + cells in haematoxylin and eosin and IHC, and disrupted induction of beige adipocyte/thermogenic genes; the levels approximated those of RT controls ( Fig. 8a–e ). The induced SMA-DTA and SMA-PPARγ fl/fl mice had normal activity, body weight and food intake, and appeared phenotypically normal ( Supplementary Fig. 8b,c , not shown) [14] . At RT, white and classical brown adipose depots and non-adipose tissues had normal weight and histological appearance, had normal vessels and did not display vascular leakage or haemorrhage, consistent with previous reports [14] ( Supplementary Fig. 8d–g ). We also repeated the Rosa26R-DTA necessity studies using the SMA-rtTA driver strain and found similar results: lower temperature, elevated sera glucose and blunted beiging as assessed by histology and beige gene expression ( Supplementary Fig. 9a–d ). We also found that SMA-rtTA-DTA mutant mice housed at RT appeared normal and had preserved body weight and food intake ( Supplementary Fig. 9e,f ). To attempt to assess whether the blunted beiging observed in vivo might be due to cell autonomous actions, we turned to ex vivo analyses. For this, we TM induced SMA-PPARγ fl/fl mice and then isolated and cultured SV cells in beige adipogenic conditions. Similar to the in vivo setting, beige adipocyte formation was disrupted with blunted expression of beige markers, indicating a potential cell autonomous effect ( Fig. 8f ). 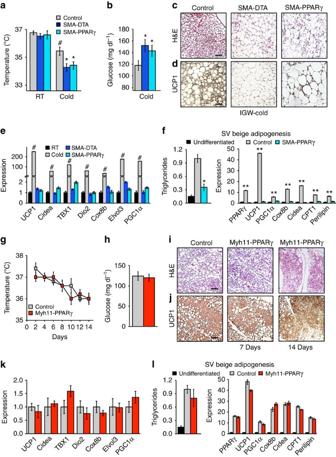Figure 8: SMA+ mural cells are required for beige adipocyte formation. (a–d) Two-month-oldSMA-CreERT2; PPARγfl/florSMA-CreERT2; R26RDTAwere administered one dose of TM for 2 consecutive days. Mice were then randomized to RT or cold exposed. Seven days later, mice were analysed for beige adipocyte formation by the following: rectal temperature (a), blood glucose levels (b), haematoxylin and eosin (H&E) staining (c), UCP1 IHC (d) and mRNA expression of beige and thermogenic markers (e). (f) SV cells were isolated from TM-induced SMA-CreERT2or SMA-CreERT2; PPARγfl/flmice and incubated in beige adipogenic culture conditions. Triglyceride content and mRNA expression of beige and thermogenic genes were analysed to determine adipocyte differentiation. Data are means±s.e.m. (n=4 mice per group replicated thrice). Studentst-test, *P-value <0.05, SMA-CreERT2; PPARγfl/florSMA-CreERT2; R26RDTAcompared with control. Studentst-test, #P-value <0.05, cold control compared with RT control. Studentst-test, **P-value <0.01, control compared with undifferentiated SV cells. (g–k) Two-month-old Myh11-PPARγmale mice were administered one dose of TM for 2 consecutive days. Mice were then randomized to RT or cold for 1 or 2 weeks. Mice were analysed for beige adipocyte formation by the following: rectal temperature (g), blood glucose levels (h), H&E staining (i), UCP1 IHC (j) and mRNA expression of beige markers (k). Data are means±s.e.m. (n=4 mice per group replicated thrice. Scale bar, 100 μm. (l) SV cells were isolated from TM-induced Myh11CreERT2; PPARγfl/flmice and incubated in adipogenic conditions. Triglyceride content and mRNA expression of beige and thermogenic genes were analysed to determine adipocyte differentiation. Data are means±s.e.m. (n=4 mice per group replicated twice). Figure 8: SMA+ mural cells are required for beige adipocyte formation. ( a – d ) Two-month-old SMA-Cre ERT2 ; PPARγ fl/fl or SMA-Cre ERT2 ; R26R DTA were administered one dose of TM for 2 consecutive days. Mice were then randomized to RT or cold exposed. Seven days later, mice were analysed for beige adipocyte formation by the following: rectal temperature ( a ), blood glucose levels ( b ), haematoxylin and eosin (H&E) staining ( c ), UCP1 IHC ( d ) and mRNA expression of beige and thermogenic markers ( e ). ( f ) SV cells were isolated from TM-induced S MA-Cre ERT2 or S MA-Cre ERT2 ; PPARγ fl/fl mice and incubated in beige adipogenic culture conditions. Triglyceride content and mRNA expression of beige and thermogenic genes were analysed to determine adipocyte differentiation. Data are means±s.e.m. ( n =4 mice per group replicated thrice). Students t -test, * P -value <0.05, S MA-Cre ERT2 ; PPARγ fl/fl or SMA-Cre ERT2 ; R26R DTA compared with control. Students t -test, # P -value <0.05, cold control compared with RT control. Students t -test, ** P -value <0.01, control compared with undifferentiated SV cells. ( g – k ) Two-month-old Myh11-PPAR γ male mice were administered one dose of TM for 2 consecutive days. Mice were then randomized to RT or cold for 1 or 2 weeks. Mice were analysed for beige adipocyte formation by the following: rectal temperature ( g ), blood glucose levels ( h ), H&E staining ( i ), UCP1 IHC ( j ) and mRNA expression of beige markers ( k ). Data are means±s.e.m. ( n =4 mice per group replicated thrice. Scale bar, 100 μm. ( l ) SV cells were isolated from TM-induced Myh11Cre ERT2 ; PPAR γ fl/fl mice and incubated in adipogenic conditions. Triglyceride content and mRNA expression of beige and thermogenic genes were analysed to determine adipocyte differentiation. Data are means±s.e.m. ( n =4 mice per group replicated twice). Full size image A potential issue of deleting PPARγ in SMA + mural cells could be changes in vascular function or integrity, which could alter cold responses and beiging. To pursue this notion we turned to the Myh11-Cre ERT2 mice, because in flow cytometry studies the Myh11-Cre ERT2 ; RFP marked roughly the same percentage (8–13%) of white adipose tissue vascular-residing mural cells as did the SMA drivers, and because Myh11 is also expressed in many other mural compartments and muscle cells throughout the body ( Supplementary Fig. 6 ). Nevertheless, the Myh11-Cre ERT2 ; RFP had a much lower beige adipocyte fate-mapping potential than SMA driver mice ( Figs 1 and 2 , and Supplementary Figs 1 and 2 ). Therefore, using the Myh11-Cre ERT2 driver to alter PPARγ function might allow discrimination between possible changes in vascular function, presumably present in roughly equal amounts in the Myh11 and SMA driver settings. We incorporated the PPARγ fl/fl allele with Myh11-Cre ERT2 , to generate Myh11-Cre ERT2 ; PPARγ mice and induced PPARγ deletion by administering one dose of TM for 2 consecutive days. After washout, we housed these mice in the cold for 7 and 14 days, and our analyses indicated that cold-induced beiging and cold-induced physiological responses were unchanged. For example, body temperatures and sera glucose levels were similar between controls and mutants ( Fig. 8g,h ). Histological, IHC and molecular analyses indicated that beige adipocyte formation was unchanged between controls and mutants ( Fig. 8i–k ). Myh11-Cre ERT2 ; PPARγ -deleted mice appeared phenotypically normal and had similar body weight and adipose tissue weight at RT. We also did not observe any vasculature abnormalities or leak within the white adipose depots (not shown). We also analysed ex vivo beige adipogenic potential and isolated SV cells from TM-induced control and Myh11-Cre ERT2 ; PPARγ mice. We cultured the cells to confluence, incubated them in beige adipogenic conditions and quantified triglyceride accumulation and beige marker expression. These studies indicated that beige adipogenesis was relatively normal; both triglyceride content and mRNA levels of beige adipocyte markers were similar in control and mutant cells ( Fig. 8l ). Cold-induced beige adipocytes convert glucose and fatty acids to heat, thereby potentially increasing energy expenditure [26] , [48] , [49] , [50] , [51] , [52] . These beige cellular furnaces could help address the widespread and conjoined obesity and diabetes epidemics [53] , [54] , [55] . Stimulating beige adipocyte formation and function may therefore lead to improved glucose homeostasis, increased metabolic rate and lower adiposity, and some clinical studies support this notion [56] , [57] , [58] , [59] . This therapeutic potential has been limited, because the origins of beige adipocytes are not well understood, because the precise cellular source of the beige phenomenon is controversial and because additional tools to mark and manipulate beige progenitors are needed. Our data, based on a series of adipocyte, muscle and mural cell Cre and inducible Cre genetically modified mouse strains suggest that white adipose tissue-resident mural cells are an important cellular source of cold-induced beige adipocytes. Several mural-marking mice displayed fate mapping into beige adipocytes and two independent inducible SMA -based strains, SMA-Cre ERT2 and SMA-rtTA , appeared suited to explore and delineate cold-induced beige biology. For example, the majority of cold-induced beige adipocytes seemed to derive from the SMA -marked sources. Although neither white nor beige adipocytes appeared to express endogenous SMA , or SMA-Cre ERT2 - or SMA-rtTA- driven RFP (on activation of the reporter), mural cells did and in a restricted manner. When we disrupted SMA -expressing cell function, by inhibiting adipocyte differentiation (deleting PPARγ ) or with a cell-killing strategy (activating DTA ) in SMA-Cre ERT2 cells and using SMA-rtTA to activate DTA , beiging was impaired in vivo and ex vivo . In these three mutant mouse strains, not only was beige adipocyte formation diminished but also the mutant mice were unable to appropriately defend body temperature and had elevated glucose levels. However, it is plausible that some of these effects on blood glucose and temperature could stem from roles of SMA-Cre ERT2 - and SMA-rtTA-expressing cells in adipose mural cells that did not have progenitor potential and in non-adipose tissues such as cardiac and skeletal muscles, as both these drivers mark these tissues ( Fig. 1 and Supplementary Figs 5 and 6 ) [21] . For example, the SMA-DTA models could have increased skeletal muscle cell death, which could lower body temperature due to impaired or lack of shivering (muscle contraction). Further, glucose uptake could also be diminished due to muscle atrophy. Nevertheless, histologically, these tissues appeared normal, the mice appeared healthy and had normal food intake and activity, and at RT the strains did not appear to have an altered phenotype. To attempt to control for some of these non-autonomous concerns, we also altered PPARγ function using the Myh11-Cre ERT2 driver; these mice had normal beiging, normal blood glucose levels and were able to defend their body temperature. Nonetheless, further characterization is needed to further delineate potential ‘side effects’ of ablating SMA + cells in all SMA driver-expressing tissues. The data in this study in concert with other reports indicate that white and beige adipocyte progenitors may have common features such as lineage origin, cell compartment locality and others. For example, the SMA drivers’ fate map into white adipocytes under the influence of some stimuli such as RT and into beige adipocytes under other conditions such as cold exposure. This raises an interesting scenario in which cold exposure first triggers the SMA -marked mural cells to undergo formation of white adipocytes that then convert to a beige adipocyte phenotype. This possibility is in line with the conventional hypothesis of a white to beige transdifferentiation. However, this is not yet clear whether the same SMA -marked cell can give rise to both white and beige adipocytes or to only one cell type. Further studies and genetic tools are needed to tease apart the functions and relationships of white and beige progenitors. In addition to SMA we found that other mural cell Cre/inducible Cre drivers marked cold-induced beige adipocytes. In agreement with Spiegelman and colleagues [11] , we observed that Myh11 + cells fate mapped into 12% of beige adipocytes after 2 weeks of cold exposure. AdipoTrak also marked the cold-induced beiging process as did NG2 and SM22 ; however, these tools have caveats. AdipoTrak in the unsuppressed state marks the mural progenitors, but also the forming adipose lineage and mature adipocytes. These issues can be overcome when combining Dox suppression/release and H2B-GFP marking, the labeling of actively proliferating cells in the mural compartment. With this method, we found that mural progenitor marking is relatively restricted but this restriction evolves under the influence of cold temperatures to include fate mapping into beige adipocytes. This supports the mural progenitor hypothesis and the notion that during lineage specification amplification of the compartment is present. NG2-Cre ERT2 has issues in subcutaneous depots, as it marked both the progenitor and adipocyte compartment, potentially masking the source of cold-induced beige adipocytes. Of note, in subcutaneous depots 100% of white adipocytes were marked, but only about 50% of beige adipocytes were marked after cold exposure, consistent with the possibility that non-adipocytes are key sources of cold-induced beiging. Similar outcomes (100% white adipocyte marking to 45% beige adipocyte marking post cold) in retroperitoneal depots of Myf5-Cre; RFP mice amplify this notion. In visceral depots, NG2-Cre ERT2 marking appeared to have relative restriction to the mural progenitor compartment, not marking white mature adipocytes, and did fate map into cold-induced beige adipocyte formation. The SM22-Cre strain labelled a majority of beige adipocytes and the mural perivascular compartment; however, this tool suffers from the lack of inducibility of straight Cre tool/systems; active and historically SM22-Cre -expressing cells will be labelled. This cell marking system is likely to be inappropriate for fate mapping because of the inability to determine when and where SM22 is expressed (stem, progenitor, mature adipocyte and embryonic timing and so on). The fact that a wide range of independently derived mural marking strains (for example, AdipoTrak , SM22-Cre , NG2-Cre ERT2 , Myh11-Cre ERT2 , SMA-Cre ERT2 and SMA-rtTA ) fate map into cold-induced beiging indicates that mural cells are a beige progenitor source. However, the strains were expressed in common and independent sets of adipose depot mural cells and the endogenous proteins also appeared to label distinct populations of mural cells. This heterogeneity may in part account for why the drivers had different fate-mapping efficiencies. Potential insight into the relationship of the different murals may be gleaned from the increase in beige adipocyte marking percentage of the Myh11 strain when comparing 1 week with 2 weeks of cold exposure. This may potentially identify an evolution of the marked cells during this time frame. More extensive lineage studies are needed to tease apart the relationship between the various mural markers and the beige progenitor mural marker signature. The development of new genetic tools may foster the ability to dissect the relevant cell types and specification steps that underlie formation of beige adipocytes. Taken together, studies support the notion that mural cells are an important source of cold-induced beiging, and that inducible SMA -based engineered mice, SMA-Cre ERT2 or SMA-rtTA , are appropriate strains to study cold-induced beige adipocyte formation and function [8] , [11] , [51] , [52] . These mouse strains and derivatives thereof may enable identification and isolation of the beige progenitors and their descendants, as well as delineation of signals and mechanisms that control cold-inducible beige behaviour—essential steps on the road to therapeutic manipulation. Animals All animals were maintained under the ethical guidelines of the UT Southwestern Medical Center Animal Care and Use Committee according to NIH guidelines. Mice were housed in a 12:12 light:dark cycle at 23 °C, and chow and water were provided ad libitum . Adiponectin-Cre ERT2 (Stock 024671), Myf5-Cre (Stock 007893), SM22-Cre (Stock 017491), Myh11-Cre ERT2 (Stock 019079), NG2-Cre ERT2 (Stock 008538), PPARγ fl/fl (Stock 004584), Rosa26R DTA (Stock 006331) and Rosa26R RFP (Stock 007914) mice were obtained from the Jackson Laboratory. AdipoTrak and aP2-Cre ERT2 were previously described [11] . Dr Eric Olson generously provided Myogenin-Cre and UCP1-Cre ERT2 mice. Dr Pierre Chambon generously provided SMA-Cre ERT2 mice. Dr Beverly Rothermel generously provided SMA-rtTA mice . Drs Sean Morrison and Bill Richardson generously provided the PDGFRα-Cre ERT2 mice. We performed experiments on 2-month-old males, unless specific ages were specified. All Cre mouse strains were maintained on a C57BL/6J and 129SV mixed background. Pure C57BL/6J 2-month-old male mice were purchased from Jackson Laboratories. Cre recombination was induced by administering TM dissolved in sunflower oil (Sigma, 100 mg kg −1 interperitoneal injection) on 2 consecutive days. Twenty-four hours post TM injection is considered a pulse. rtTA activation was induced by Dox (0.5 mg ml −1 in 1% sucrose) provided in the drinking water and protected from light, and it was changed every 2–3 days. For cold studies, mice were placed in a 6 °C cold metabolic chamber for 7–14 days. After recombination was induced, mice were randomized to RT or cold exposed for 7–14 days. We performed experiments on mice after a 48-h TM washout period, a week TM washout period and a 2-week TM washout period. No animals were excluded from any experiments unless mice displayed wounds from fighting. Histology Haematoxylin and eosin staining was carried out on paraffin sections using standard methods. Adipose tissues were fixed in formalin overnight, dehydrated, embedded in paraffin and sectioned with a microtome at 5–8 μm thicknesses. Immunostaining was performed in either paraffin sections or cryostat sections (5–8 μm) of tissues freshly embedded in optical coherence tomography [13] . Briefly, samples were pre-incubated with permeabilization buffer (0.3% Triton X-100 in PBS) for 30 min at RT and then incubated sequentially with primary antibody (4 °C, overnight) and secondary antibody (2 h at RT), all in blocking buffer (5% normal donkey serum in 1 × PBS). Antibodies used for immunostaining are as follows: rabbit-anti-UCP1 (1:200, Abcam), mouse-anti-RFP (1:100, Clontech), rat-anti-PECAM (1:200, BD Biosciences), rabbit-anti-α-SMA (1:200, Sigma) and goat-anti-Perilipin (1:200, BD Biosciences). For negative control subjects, primary antibody was replaced with 5% normal donkey serum. Secondary antibodies including cy3 donkey anti-mouse, cy2 donkey anti-rabbit and cy2 donkey anti-rat were from Jackson ImmunoResearch. All secondary antibodies were used at a 1:500 dilution. Lipid was stained with LipidTOX Green (1:100, Life Technologies). Immunostaining images were collected on a Zeiss LSM500 confocal microscope, an Olympus IX70 inverted microscope or an Olympus upright BX40 microscope. All experimental and control images of the immunofluorescence data were collected using identical imaging settings. Paraffin-embedded tissues were sectioned with a Microm HM 325 microtome. Cryostat sectioning was performed with a Microm HM505 E cryostat. Co-localization quantification For quantification of images, two independent observers assessed three random fields in ten random sections from at least three mice per cohort. NIH Image J software using the JACoP [60] (Just Another Colocalization Plugin) extension was used to quantify co-localization. First, the total area of UCP1 immunostaining was calculated. Next, the area of co-localized UCP1 immunostaining and RFP (for all drivers) was calculated. To derive the total percentage of co-localization, the per cent co-localization between UCP1 immunostaining and RFP was divided by the total area of UCP1 immunostaining. To identify SMA-Cre ERT2 ; RFP expression in mature adipocytes, mice were administered one dose of TM for 2 consecutive days. Subcutaneous and visceral adipose depots were isolated and adipocytes were fractioned by floatation. Adipocytes were stained with LipidTOX (Life Technologies) and DAPI (4,6-diamidino-2-phenylindole) to visualize intact adipocytes. For quantification of images, two independent observers assessed three random fields in ten random sections from at least three mice per cohort. Positivity was assessed by LipidTox+, DAPI+ and RFP+. Stromal vascular fractionation The SV cells were isolated [13] . Briefly, we pooled subcutaneous (inguinal and periscapular) white adipose tissues for fractionation, unless indicated otherwise. After 2 h of slow shaking in isolation buffer (100 mM HEPES pH 7.4, 120 mM NaCl, 50 mM KCl, 5 mM glucose, 1 mM CaCl2, 1.5% BSA) containing 1 mg ml −1 collagenase at 37 °C, the digest was pipetted up and down a few times for better dissociation. The suspension was then spun at 800 g for 10 min; the resultant floating layer was the adipocyte layer and the pellet was a crude SV fraction. The floating adipocyte layer was washed in 1 × PBS, spun at 800 g for 5 min and the solution was removed from below. The pellet was then resuspended in erythrocyte lysis buffer (0.83% NH 4 Cl in H 2 O) for 8 min and spun at 800 g for 5 min. The pellet was washed once in 1 × PBS, resuspended and passed through 30 μm mesh. Cell culture Isolated SV cells were cultured in DMEM supplemented with 10% fetal bovine serum (FBS). White adipogenesis was induced by treating confluent cells with DMEM containing 10% FBS, insulin (0.5 μg ml −1 ), dexamethasone (5 μM) and isobutylmethylxanthine (0.5 mM) [11] . Beige adipogenesis was induced by treating confluent cells with DMEM containing 10% FBS, insulin (0.5 μg ml −1 ), dexamethasone (5 μM), isobutylmethylxanthine (0.5 mM), troglitazone (1 μM), 5 nM indomethacin and T3 (2 nM) [44] . To induce thermogenic genes, cells were treated with 10 μM forskolin for 4 h and harvested to collect mRNA [55] . Triglyceride accumulation assay was performed using a kit from ZenBio [61] following the manufacturer’s protocol. To induce SMA-Cre ERT2 ; RFP recombination ex vivo , adipocytes were isolated from 2-month-old uninduced SMA-Cre ERT2 ; RFP male mice. TM (1 μM) was then administered ex vivo for 24 h and the floated adipocytes were fluorescence microscopically assessed for RFP and lipid (LipidTox, Life Technologies). Flow cytometry and sorting SV cells were isolated [11] and washed, centrifuged at 800 g for 5 min and analysed with a FACScans analyser or sorted with a BD FACS Aria operated by the UT Southwestern Flow Cytometry Core. Data analysis was performed using BD FACS Diva software. For RFP+ sorting, live SV cells from young 2-month-old R26R RFP mice were stained with propidium iodide (1 mg ml −1 ) to exclude dead cells and sorted based on native fluorescence (RFP). The SV cells from control mice were used to determine background fluorescence levels. The dissociated SV cells were also analysed for mural and perivascular markers by flow cytometry. Briefly, SV cells were incubated with primary antibodies on ice for 30 min and then washed twice with the staining buffer and incubated with secondary antibody for another 30 min on ice before flow cytometric analysis. Quantitative real-time PCR Total RNA was extracted using TRIzol (Invitrogen) from either mouse tissues or cells. Complementary DNA synthesis was performed using Superscript III reverse transcriptase (Invitrogen) using 1 μg of RNA [13] . Gene expression was analysed using Power SYBR Green PCR Master Mix with ABI 7500 Real-Time PCR System. qPCR values were normalized by 18s rRNA expression. Primer sequences are available on request. Metabolic phenotyping experiments Temperature was monitored daily using a rectal probe (Physitemp) [62] . Briefly, the probe was lubricated with glycerol and was inserted 1.27 cm (1/2 inch) and temperature was measured when stabilized. Glucose monitoring, that is, blood glucose levels were measured with a Contour glucometer (Bayer). Statistical analysis Statistical significance assessed by two-tailed Student’s t -test. Data are shown as means and error bars indicate s.e.m. Studies were performed on two or three independent cohorts and were performed on three to four mice per group unless specified. Sample size was determined using previous experimental studies for fate mapping and metabolic assessment. Mice were randomized to the cold temperature or RT in a blinded manner. How to cite this article: Berry, D. C. et al. Mouse strains to study cold-inducible beige progenitors and beige adipocyte formation and function. Nat. Commun. 7:10184 doi: 10.1038/ncomms10184 (2016).